Pseudomonas aeruginosaeradicatesStaphylococcus aureusby manipulating the host immunity Young cystic fibrosis (CF) patients’ airways are mainly colonized by Staphylococcus aureus , while Pseudomonas aeruginosa predominates in adults. However, the mechanisms behind this infection switch are unclear. Here, we show that levels of type-IIA-secreted phospholipase A2 (sPLA2-IIA, a host enzyme with bactericidal activity) increase in expectorations of CF patients in an age-dependent manner. These levels are sufficient to kill S. aureus , with marginal effects on P. aeruginosa strains. P. aeruginosa laboratory strains and isolates from CF patients induce sPLA2-IIA expression in bronchial epithelial cells from CF patients (these cells are a major source of the enzyme). In an animal model of lung infection, P. aeruginosa induces sPLA2-IIA production that favours S. aureus killing. We suggest that sPLA2-IIA induction by P. aeruginosa contributes to S. aureus eradication in CF airways. Our results indicate that a bacterium can eradicate another bacterium by manipulating the host immunity. Cystic fibrosis (CF) is a lethal autosomal, recessive inherited disease that commonly affects Caucasians [1] , [2] . This disease is due to mutation of CF transmembrane conductance regulator (CFTR) gene [3] , [4] that encodes a protein channel in epithelial cells where it regulates the luminal secretion of chloride and water transport. The F508del-CFTR is the most frequent mutation in CFTR present in CF patients [5] . Pulmonary disease in CF is the major problem that determines the life span and life quality of patients [6] and contributes to 80–95% death of CF patients [7] , [8] , [9] . In the lungs, mutations of CFTR cause depletion of airway surface liquid and mucus dehydration, which provide an appropriate niche for chronic bacterial infection by opportunistic pathogens. Bacterial airways infection varies significantly with the age of patients and Staphylococcus aureus (SA) is the most commonly isolated bacterium from young CF patients [10] , [11] , [12] . With the increase of age of patients, Pseudomonas aeruginosa (PA) becomes predominant and in the adult patients represents over 80% of bacteria in the lung [8] , [12] , [13] . However, the mechanisms responsible for this age-related infection switch from SA to PA remained unclear. We hypothesized that a selective elimination of SA in CF airways by a host molecule endowed with antibacterial activity might be involved in the infection switch from SA to PA. According to our hypothesis, the levels of this molecule would increase with age of CF patients and PA infection leading to progressive elimination of SA from airways. Among the host molecules endowed with antibacterial properties, antimicrobial peptides (AMPs) play a key role in natural host defense toward invading pathogens [14] , [15] , [16] . AMPs are ubiquitous, gene-encoded natural ‘antibiotics’ including cationic peptides, defensins and some secreted phospholipases A2 (sPLA2s) [14] , [17] . PLA2s represent a superfamily of intracellular and secreted enzymes, which hydrolyse membrane phospholipids of eukaryotic and prokaryotic cells [15] and participate in a variety of processes such as inflammation and host defense mechanisms [18] . Among mammalian PLA2s, type-IIA-secreted PLA2 (sPLA2-IIA) has been shown to exert a potent bactericidal effect [14] , [19] . Gram-positive bacteria are much more sensitive to sPLA2-IIA than Gram-negative bacteria due to higher affinity of sPLA2-IIA to the cell walls of Gram-positive bacteria [14] , [17] . Selective hydrolysis of bacterial membrane phospholipids represents the critical step of bactericidal action of sPLA2-IIA [20] . This enzyme is the most potent bactericidal agent produced by mammals [17] and is, for example, the principal bactericidal molecule for SA in human tears [21] . Here, we show that sPLA2-IIA is present in expectorations of CF patients at levels sufficient to kill SA with a limited effect on PA. The levels of enzyme increase with the age of CF patients. Both clinical isolates of SA freshly collected from CF patients and SA laboratory strains are killed efficiently by recombinant human sPLA2-IIA (rhsPLA2-IIA). However, this enzyme has a limited effect on PA from both laboratory strains and isolates collected from CF patients. Most importantly, we find that PA (laboratory strains and CF isolates), but not SA, induces sPLA2-IIA expression by bronchial epithelial cells (BECs) obtained from CF patients. Using bacterial mutants, we show that the secreted toxin ExoS is the PA virulence factor involved in the induction of sPLA2-IIA expression by BECs. Studies on animal models of airways coinfection by SA and PA demonstrate the role of sPLA2-IIA in the selective airways clearance of SA compared to PA. The presence of PA in airways enhances SA clearance by increasing sPLA2-IIA production. This work thus provides a pathophysiological significance for the selectivity of sPLA2-IIA bactericidal effect towards the Gram-positive bacteria. It also indicates that a bacterium can eradicate another bacterium by manipulating the innate immunity of the host. sPLA2-IIA levels in CF airways are sufficient to kill SA Given that sPLA2-IIA is known to exert potent bactericidal effects against Gram-positive bacteria [14] , [17] , we examined at first the presence of this enzyme in the expectorations from CF patients. It is not possible to obtain sputum from healthy individuals. Expectorations are produced only under particular pathological conditions such as CF. Our data showed that sPLA2-IIA was present in CF expectorations and its levels significantly increased with the age of patients, reaching a plateau near the age of 15–20 years ( Fig. 1a , Supplementary Fig. 1a ). As expected, IL8 and IL1β were also detected in CF expectorations ( Supplementary Fig. 1b,c ). A weak negative correlation was observed between sPLA2-IIA and IL8 and no correlation was observed between sPLA2-IIA and IL1β levels ( Supplementary Fig. 1d,e ). 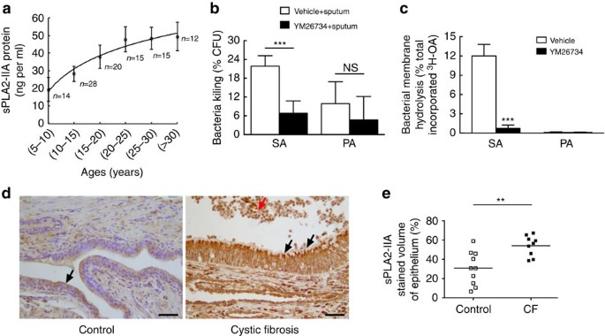Figure 1: sPLA2-IIA levels in CF airways are sufficient to kill SA. (a) sPLA2-IIA levels in expectorations at different age groups of CF patients.nindicated the number of patients per age group.n=104 total sputa. (b) Bactericidal effect of sPLA2-IIA contained in expectorations against SA (Newman strain) and PA (PAK strain). PA or SA was incubated for 2 h with CF expectorations, pretreated with or without sPLA2 inhibitor YM26734. Total c.f.u. were counted by plating on LB-agar plates. Killing effect was expressed as percentage-killed bacteria referred to PBS treatment, defined as no killing.n=104 sputa tested in each group. (c) Membrane hydrolysis of3H-oleic acid-labelled SA (3H-OA-SA) and PA (3H-OA-PA) by sPLA2-IIA contained in expectorations of CF patients. The expectorations were pretreated with YM26734 or vehicle before incubation with3H-OA-SA or3H-OA-PA.n=13 sputa tested per group (d) Airway sections obtained in a Control patient and a CF patient were stained with an antibody raised against sPLA2-IIA (brown colour) and counterstained with haematoxylin. In the Control subject, only sparse staining for sPLA2-IIA was present in the epithelium. In the CF patient, extensive staining for sPLA2-IIA was present in epithelium. Photomicrographs were representative of results obtained in 10 Controls and in nine CF patients. Black arrows: epithelial cells, red arrow: neutrophils. Scale bars, 50 μm. Original magnification: × 200. (e) Morphometric analysis of sPLA2-IIA immunostaining in the airways of Controls (white square,n=10) and of CF subjects (black square,n=9). Airway sections were immunostained for sPLA2-IIA. Morphometric analysis was performed using point counting. sPLA2-IIA positively stained volume in epithelium was significantly higher in CF versus control airways. (Pvalue=0.006). All data were presented as mean±s.e.m. **P<0.01, ***P<0.001 determined by one-way analysis of variance followed by Bonferroni multiple’s comparisons test or Student’st-test. NS, no significance. Figure 1: sPLA2-IIA levels in CF airways are sufficient to kill SA. ( a ) sPLA2-IIA levels in expectorations at different age groups of CF patients. n indicated the number of patients per age group. n =104 total sputa. ( b ) Bactericidal effect of sPLA2-IIA contained in expectorations against SA (Newman strain) and PA (PAK strain). PA or SA was incubated for 2 h with CF expectorations, pretreated with or without sPLA2 inhibitor YM26734. Total c.f.u. were counted by plating on LB-agar plates. Killing effect was expressed as percentage-killed bacteria referred to PBS treatment, defined as no killing. n =104 sputa tested in each group. ( c ) Membrane hydrolysis of 3 H-oleic acid-labelled SA ( 3 H-OA-SA) and PA ( 3 H-OA-PA) by sPLA2-IIA contained in expectorations of CF patients. The expectorations were pretreated with YM26734 or vehicle before incubation with 3 H-OA-SA or 3 H-OA-PA. n =13 sputa tested per group ( d ) Airway sections obtained in a Control patient and a CF patient were stained with an antibody raised against sPLA2-IIA (brown colour) and counterstained with haematoxylin. In the Control subject, only sparse staining for sPLA2-IIA was present in the epithelium. In the CF patient, extensive staining for sPLA2-IIA was present in epithelium. Photomicrographs were representative of results obtained in 10 Controls and in nine CF patients. Black arrows: epithelial cells, red arrow: neutrophils. Scale bars, 50 μm. Original magnification: × 200. ( e ) Morphometric analysis of sPLA2-IIA immunostaining in the airways of Controls (white square, n =10) and of CF subjects (black square, n =9). Airway sections were immunostained for sPLA2-IIA. Morphometric analysis was performed using point counting. sPLA2-IIA positively stained volume in epithelium was significantly higher in CF versus control airways. ( P value=0.006). All data were presented as mean±s.e.m. ** P <0.01, *** P <0.001 determined by one-way analysis of variance followed by Bonferroni multiple’s comparisons test or Student’s t -test. NS, no significance. Full size image We next examined the ability of sPLA2-IIA contained in CF expectorations to kill SA and PA. Our studies showed that patients’ expectorations killed SA with higher efficiency than PA and that SA killing was inhibited by pretreating expectorations with the sPLA2 inhibitor YM26734 ( Fig. 1b ). These findings were confirmed using a more specific sPLA2-IIA inhibitor RO032007A [22] and a sPLA2-IIA-neutralizing antibody [23] (which led to total abolition of SA killing by expectorations ( Supplementary Fig. 2a )). We also searched for the presence of other sPLA2s in CF expectorations by TRFIA method [24] . We detected only sPLA2-IIA and sPLA2-X ( Supplementary Fig. 2b ). However, sPLA2-X levels were not sufficient to kill SA as determined in vitro (500 ng ml −1 ; Supplementary Fig. 2c ). Finally, we tested the bactericidal activity of sPLA2-V and sPLA2-XIIA toward SA. The results showed no killing activity with these sPLA2 ( Supplementary Fig. 2c ). We also showed that these expectorations were able to hydrolyse SA membrane phospholipids and that this hydrolysis was blocked by pretreating expectorations with YM26734 ( Fig. 1c ). However, no significant PA membrane phospholipids hydrolysis was observed with these expectorations ( Fig. 1c ). These data indicated that the sPLA2-IIA present in CF expectorations was involved in the killing of SA via the hydrolysis of SA membrane phospholipids, with only marginal effect on PA. Therefore, we searched for the source of sPLA2-IIA in lungs of CF patients by using immunohistochemistry on lung explants from 10 non-CF and nine CF patients. All CF patients were infected with PA ( Supplementary Table 1 ). Non-CF patients are non-smoking individuals undergoing lung resection for peripheral lung cancer. It is not possible to obtain bronchial explants form non-infected CF patients because only CF patients with worsen conditions (high infectious status) are admitted for lung transplantation. A marked immunostaining of sPLA2-IIA was observed in all sections of bronchial explants from CF compared with non-CF patients ( Fig. 1d,e ). Positive staining was observed in surface of airway epithelial cells ( Fig. 1d , black arrows). Infiltrating neutrophils were also positively stained in explants of CF patients but were virtually absent in explants of non-CF patients ( Fig. 1d , red arrow). SA isolates of CF patients are killed by sPLA2-IIA We next compared the bactericidal effect of rhsPLA2-IIA on clinical isolates and laboratory strains of SA and PA in vitro . Remarkably, sPLA2-IIA killed efficiently all SA isolates collected from CF patients without significant effects on PA isolates ( Fig. 2a,b ). When testing laboratory strains, high concentrations (up to 10 μg ml −1 ) of rhsPLA2-IIA had only marginal bactericidal effect on all tested PA strains ( Supplementary Fig. 3a ). However, sPLA2-IIA killed all tested SA laboratory strains with an EC 50 ≤50 ng ml −1 ( Supplementary Fig. 3b ). This EC 50 value was near sPLA2-IIA levels detected in CF expectorations (around 40 ng ml −1 , Fig. 1a ). Similar bactericidal effect was observed when rhsPLA2-IIA was incubated with SA/PA mixed suspension ( Supplementary Fig. 3c ). We next examined the mechanisms by which rhsPLA2-IIA killed SA. Killing of SA was abolished by YM26734 ( supplementary Fig. 3d ). This enzyme increased the hydrolysis of SA membrane phospholipids, which was inhibited by YM26734 ( Supplementary Fig. 3e ). No significant membrane phospholipids hydrolysis was observed in antibiotics-treated or heat-killed SA, indicating that phospholipids hydrolysis was specifically due to sPLA2-IIA ( Supplementary Fig. 3f ). On the other hand, only limited hydrolysis of PA membrane phospholipids was observed even with 100 times higher sPLA2-IIA concentrations ( Supplementary Fig. 3e ). 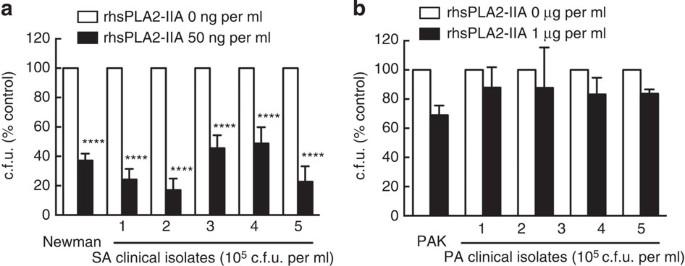Figure 2: SA isolates from CF patients are killed by rhsPLA2-IIA. Bactericidal effect of rhsPLA2-IIA against clinical isolates of SA (a) and PA (b). Newman and PAK were used as reference strains for SA and PA, respectively. Bacteria were incubated with recombinant human sPLA2-IIA (rhsPLA2-IIA, 50 ng ml−1for SA or 1 μg ml−1for PA) or PBS for 2 h. Total c.f.u. were quantified by plating on LB-agar plates. Bars graph represent survival of bacteria compared with PBS treatment. Graphs showed results of five clinical isolates of SA and PA. All data were presented as mean±s.e.m. from three independent experiments. ****P<0.0001 determined by one-way analysis of variance followed by Bonferroni multiple’s comparisons test. Figure 2: SA isolates from CF patients are killed by rhsPLA2-IIA. Bactericidal effect of rhsPLA2-IIA against clinical isolates of SA ( a ) and PA ( b ). Newman and PAK were used as reference strains for SA and PA, respectively. Bacteria were incubated with recombinant human sPLA2-IIA (rhsPLA2-IIA, 50 ng ml −1 for SA or 1 μg ml −1 for PA) or PBS for 2 h. Total c.f.u. were quantified by plating on LB-agar plates. Bars graph represent survival of bacteria compared with PBS treatment. Graphs showed results of five clinical isolates of SA and PA. All data were presented as mean±s.e.m. from three independent experiments. **** P <0.0001 determined by one-way analysis of variance followed by Bonferroni multiple’s comparisons test. Full size image sPLA2-IIA contributes to airways clearance of SA We next examined the in vivo antibacterial function of sPLA2-IIA using transgenic mice overexpressing human sPLA2-IIA (sPLA2-IIA-Tg) [25] . Increased levels of sPLA2 activity were found in bronchoalveolar lavage fluids (BALFs) from these mice compared with their littermates c57BL/6, which are naturally deficient for sPLA2-IIA (sPLA2-IIA-Wt) [25] ( Supplementary Fig. 4a ). No mortality was observed in sPLA2-IIA-Tg and sPLA2-IIA-Wt mice infected with SA at doses of 10 6 , 10 7 and 10 8 c.f.u. ( Fig. 3a–c ). But, at 10 9 c.f.u., sPLA2-IIA-Tg mice exhibited higher survival compared with sPLA2-IIA-Wt mice following SA infection ( Fig. 3d ). This finding was confirmed with another SA laboratory strain SA25923 ( Supplementary Fig. 5 ). However, at all PA doses used, no significant differences in mortality were observed between sPLA2-IIA-Tg and sPLA2-IIA-Wt mice ( Fig. 3a–d ). This suggested that sPLA2-IIA protected mice from SA infection. This protective role was further examined in mice coinfected with SA and PA (10 6 c.f.u. each). An increased elimination of SA was observed in sPLA2-IIA-Tg mice compared with their littermates, 6 and 24 h after coinfection ( Fig. 3e,f ). However, PA was cleared with almost similar velocity in sPLA2-IIA-Wt versus sPLA2-IIA-Tg mice, 6 or 24 h after coinfection ( Fig. 3e,f ). No significant difference was observed in the extent of lung inflammation without infection between sPLA2-IIA-Wt and sPLA2-IIA-Tg mice, as assessed by analysis of cell number and cytokines levels ( Supplementary Fig. 4b–e ). Infection by PA increased lung inflammation at similar levels in sPLA2-IIA-Wt and sPLA2-IIA-Tg mice ( Supplementary Fig. 4c–e ). 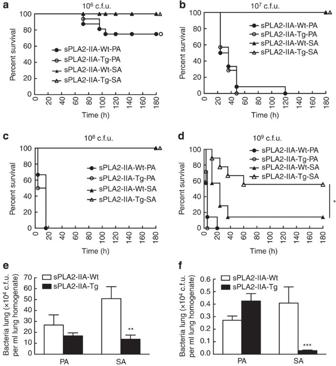Figure 3: sPLA2-IIA protects transgenic mice from SA lung infection. (a–d) Mortality of transgenic mice overexpressing human sPLA2-IIA (sPLA2-IIA-Tg) and their littermate mice (sPLA2-IIA-Wt) after lung infection with PA or SA at 106(a), 107(b), 108(c) and 109(d) c.f.u. per mouse (n≥7 per group). Data were presented as Kaplan–Meier curves. *P<0.05 compared with SA-infected sPLA2-IIA-Wt mice (Log-rank test). (e,f) Quantification of bacterial colonies in mice (n≥5 per group) lung homogenates 6 (e) or 24 h (f) after coinfection with SA and PA. Lung homogenates were plated on LB-agar plates for total bacteria quantification. All data ine,fwere presented as mean±s.e.m. **P<0.01, ***P<0.001 compared with corresponding sPLA2-IIA-Wt mice (two-way analysis of variance). Figure 3: sPLA2-IIA protects transgenic mice from SA lung infection. ( a – d ) Mortality of transgenic mice overexpressing human sPLA2-IIA (sPLA2-IIA-Tg) and their littermate mice (sPLA2-IIA-Wt) after lung infection with PA or SA at 10 6 ( a ), 10 7 ( b ), 10 8 ( c ) and 10 9 ( d ) c.f.u. per mouse ( n ≥7 per group). Data were presented as Kaplan–Meier curves. * P <0.05 compared with SA-infected sPLA2-IIA-Wt mice (Log-rank test). ( e , f ) Quantification of bacterial colonies in mice ( n ≥5 per group) lung homogenates 6 ( e ) or 24 h ( f ) after coinfection with SA and PA. Lung homogenates were plated on LB-agar plates for total bacteria quantification. All data in e , f were presented as mean±s.e.m. ** P <0.01, *** P <0.001 compared with corresponding sPLA2-IIA-Wt mice (two-way analysis of variance). Full size image PA stimulates sPLA2-IIA production leading to SA killing We next examined whether endogenously produced sPLA2-IIA exerts a role in SA clearance in airways. Given that mice naturally exhibit very low sPLA2-IIA expression in the lungs [25] , [26] , we used guinea pigs as animal model known to produce high pulmonary levels of sPLA2-IIA (refs 17 , 27 ). At first, we examined the effect of PA and SA (5 × 10 6 c.f.u. each) on sPLA2-IIA expression in guinea pigs lungs. The results showed that intratracheal instillation of PA alone or in combination with SA to guinea pigs increased the levels of sPLA2 activity in BALFs of these animals, while SA had only a limited effect ( Fig. 4a ). This activity was almost totally abolished by pretreating BALFs with YM26734 ( Supplementary Fig. 6a ). Next, guinea pigs were infected intratracheally with PA and SA separately or in combination at various loads and ratio and then bacterial loads were analysed in BALs 24 h after coinfection. At 5 × 10 6 c.f.u. of PA or SA, SA was almost undetectable ( Supplementary Fig. 6b ). At 5 × 10 7 c.f.u. of PA and SA (1:1 ratio), most animals died within 24 h after coinfection ( Supplementary Fig. 6c ). In another set of experiments, animals were infected with 5 × 10 6 c.f.u. of PA and 5 × 10 7 c.f.u. of SA separately or in combination (1:10 ratio). In these conditions, we observed a significant decrease of SA loads in BALs from animals coinfected with PA compared with BALs from animals infected with SA alone. However, PA loads in BALs were similar in the presence or absence of SA ( Fig. 4b ). 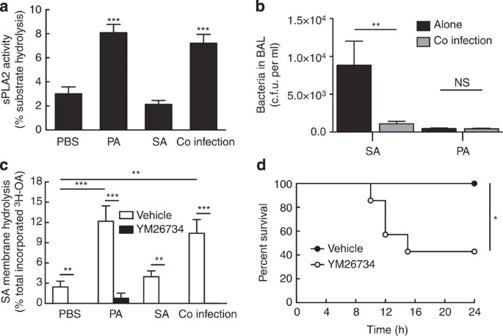Figure 4: PA-induced sPLA2-IIA participates to SA clearance in airways. (a) sPLA2 activity assay in BALFs from non-infected (PBS), PA and/or SA-infected animals (n≥3 per group). sPLA2 activity was measured using3H-OA-labelledE. colimembrane as substrate. (b) Bacterial loads in BALs from SA and/or PA intratracheally infected animals (n≥5 per group). BALs were plated on LB-agar plates for c.f.u. counting. (c) Membrane hydrolysis of3H-OA-labelled SA (3H-OA-SA) by sPLA2-IIA contained in BALFs from PBS, PA and/or SA-infected animals. BALFs were pretreated with 10 μM YM26734 or vehicle before incubation with3H-OA-SA. (d) Effect of YM26734 on mortality of guinea pigs coinfected intratracheally with SA and PA (n=3 per group). Animals were pretreated by YM76234 or vehicle before bacterial infection. Data were presented as Kaplan–Meier curves (*P<0.05, Log-rank test). Data ina–cwere shown as mean±s.e.m. **P<0.01, ***P<0.001 determined by one-way analysis of variance, followed by Bonferroni multiple’s comparisons test. *P<0.05 compared with SA-infected sPLA2-IIA-Wt mice (Log-rank test). Figure 4: PA-induced sPLA2-IIA participates to SA clearance in airways. ( a ) sPLA2 activity assay in BALFs from non-infected (PBS), PA and/or SA-infected animals ( n ≥3 per group). sPLA2 activity was measured using 3 H-OA-labelled E. coli membrane as substrate. ( b ) Bacterial loads in BALs from SA and/or PA intratracheally infected animals ( n ≥5 per group). BALs were plated on LB-agar plates for c.f.u. counting. ( c ) Membrane hydrolysis of 3 H-OA-labelled SA ( 3 H-OA-SA) by sPLA2-IIA contained in BALFs from PBS, PA and/or SA-infected animals. BALFs were pretreated with 10 μM YM26734 or vehicle before incubation with 3 H-OA-SA. ( d ) Effect of YM26734 on mortality of guinea pigs coinfected intratracheally with SA and PA ( n =3 per group). Animals were pretreated by YM76234 or vehicle before bacterial infection. Data were presented as Kaplan–Meier curves (* P <0.05, Log-rank test). Data in a – c were shown as mean±s.e.m. ** P <0.01, *** P <0.001 determined by one-way analysis of variance, followed by Bonferroni multiple’s comparisons test. * P <0.05 compared with SA-infected sPLA2-IIA-Wt mice (Log-rank test). Full size image This prompted us to investigate the effect of these BALFs on the hydrolysis of SA membrane phospholipids, which represents the key step in bacterial killing by sPLA2-IIA. BALFs from guinea pigs infected with PA alone or coinfected with PA and SA induced significant phospholipid hydrolysis of SA membranes, compared with that from non-infected or SA-infected animals ( Fig. 4c ). This hydrolysis was abrogated by pretreating BALFs with YM26734 before incubation with SA ( Fig. 4c ). In addition, our previous studies have shown that lipopolysaccharide (LPS) from PA induced an increased production of sPLA2-IIA in guinea pigs lungs [17] , [27] . Here, we incubated SA or PA laboratory strains with lung homogenates from PA LPS-treated guinea pigs. The results revealed a trend of increased SA killing by these homogenates compared with homogenates from saline-treated guinea pigs and addition of YM26734 reduced this killing ( Supplementary Fig. 6d ). However, no difference was observed in PA killing by lung homogenates from both LPS- and saline-treated guinea pigs ( Supplementary Fig. 6e ). Interestingly, intratracheal instillation of YM26734 before PA/SA coinfection of guinea pigs significantly increased animal mortality ( Fig. 4d ). YM26734 alone had no effect on animal mortality ( Supplementary Fig. 6f ) or inflammation ( Supplementary Fig. 6g ). PA induces sPLA2-IIA expression in CF epithelial cells Our data showing that BECs were a main source of sPLA2-IIA in bronchial explants of CF patients ( Fig. 1d ) prompted us to examine the effect of PA and SA on sPLA2-IIA expression by the BEC line IB3-1 bearing the F508del-CFTR mutation [28] . All tested PA strains significantly induced sPLA2-IIA expression in IB3-1 cells in parallel to IL8 secretion ( Fig. 5a , Supplementary Fig. 7a ). However, none of the tested SA strains stimulated sPLA2-IIA expression ( Fig. 5b ). Although not all of SA strains induced IL8 secretion, all tested SA strains induced higher levels of IL6 secretion than PA strain PAK, used as control ( Supplementary Fig. 7b,c ). Similarly, CF clinical isolates of PA also induced sPLA2-IIA expression by IB3-1 cells in contrast to SA isolates, which had no effect on this expression ( Fig. 5c ). As observed with laboratory strains, PA clinical isolates induced IL8 secretion, while SA isolates had limited effect ( Supplementary Fig. 7d ). But SA isolates increased IL6 production ( Supplementary Fig. 7e ). 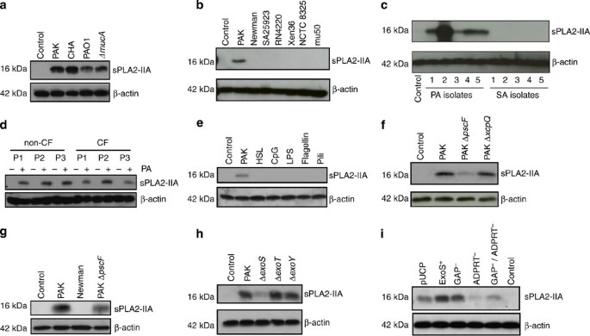Figure 5: PA toxin ExoS stimulates sPLA2-IIA expression in CF epithelial cells. (a) Western blot analysis of sPLA2-IIA expression in IB3-1 BECs after infection with different strains of PA. (b) Western blot analysis of sPLA2-IIA expression in IB3-1 cells after infection with different strains of SA. Cells were infected with PAK wild-type parental strain as positive control. (c) Western blot analysis of sPLA2-IIA expression in IB3-1 after infection with 5 clinical isolates of PA and SA collected from CF patients, respectively. (d) Western blot analysis of sPLA2-IIA expression in human primary BECs from three different non-CF and CF patients (P1–P3). Cells were either infected with PAK strain (PA) or uninfected. (e) Western blot analysis of sPLA2-IIA expression in IB3-1 cells after incubation with different preparations of PA pathogen-associated molecular patternss including LPS, flagellin, pili, CpG and HSL. (f) Western blot analysis of sPLA2-IIA expression in IB3-1 cells after infection with mutant of PAK deficient for type-T3SS (ΔpscF) or type 2 secretion system (ΔxcpQ). Cells were infected with PAK wild-type parental strain as positive control. (g) Western blot analysis of sPLA2-IIA expression in pBECs collected from CF patients after infection with SA, PA and T3SS-deficient strain of PA (ΔpscF). (h) Western blot analysis of sPLA2-IIA expression in IB3-1 cells after infection with mutants of PAK deficient for toxins ExoS (ΔexoS), ExoT (ΔexoT) and ExoY (ΔexoY). Cells were infected with PAK wild-type parental strain as positive control. (i) sPLA2-IIA expression in IB3-1 cells infected with PA103ΔUΔT strain in which different mutants of ExoS were introduced: pUCP (empty vector), ExoS+(wild-type toxin), GAP−(ExoS mutant in arginine 146), ADPRT−(ExoS mutant in glutamic acid 379 and 381) and double mutant GAP−/ADPRT−. Immunoblots shown were representative results from at least three independent experiments. Full blots are available inSupplementary Fig. 9. Figure 5: PA toxin ExoS stimulates sPLA2-IIA expression in CF epithelial cells. ( a ) Western blot analysis of sPLA2-IIA expression in IB3-1 BECs after infection with different strains of PA. ( b ) Western blot analysis of sPLA2-IIA expression in IB3-1 cells after infection with different strains of SA. Cells were infected with PAK wild-type parental strain as positive control. ( c ) Western blot analysis of sPLA2-IIA expression in IB3-1 after infection with 5 clinical isolates of PA and SA collected from CF patients, respectively. ( d ) Western blot analysis of sPLA2-IIA expression in human primary BECs from three different non-CF and CF patients (P1–P3). Cells were either infected with PAK strain (PA) or uninfected. ( e ) Western blot analysis of sPLA2-IIA expression in IB3-1 cells after incubation with different preparations of PA pathogen-associated molecular patternss including LPS, flagellin, pili, CpG and HSL. ( f ) Western blot analysis of sPLA2-IIA expression in IB3-1 cells after infection with mutant of PAK deficient for type-T3SS (Δ pscF ) or type 2 secretion system (Δ xcpQ ). Cells were infected with PAK wild-type parental strain as positive control. ( g ) Western blot analysis of sPLA2-IIA expression in pBECs collected from CF patients after infection with SA, PA and T3SS-deficient strain of PA (Δ pscF ). ( h ) Western blot analysis of sPLA2-IIA expression in IB3-1 cells after infection with mutants of PAK deficient for toxins ExoS (Δ exoS ), ExoT (Δ exoT ) and ExoY (Δ exoY ). Cells were infected with PAK wild-type parental strain as positive control. ( i ) sPLA2-IIA expression in IB3-1 cells infected with PA103ΔUΔT strain in which different mutants of ExoS were introduced: pUCP (empty vector), ExoS + (wild-type toxin), GAP − (ExoS mutant in arginine 146), ADPRT − (ExoS mutant in glutamic acid 379 and 381) and double mutant GAP − /ADPRT − . Immunoblots shown were representative results from at least three independent experiments. Full blots are available in Supplementary Fig. 9 . Full size image We also investigated whether increase in sPLA2-IIA expression in BECs was due to CFTR mutations using primary BECs (pBECs) from three different CF and non-CF patients. In basal conditions, pBECs from both CF and non-CF patients had no detectable sPLA2-IIA expression ( Fig. 5d ). However, this expression increased after PA infection but its levels remained similar in both cells types ( Fig. 5d ). This suggested that, in primary CF BECs, CFTR mutations have no effect on sPLA2-IIA expression that was clearly induced by PA infection. PA induces sPLA2-IIA expression via T3SS-dependent process We then searched for the virulence factors of PA involved in sPLA2-IIA expression by BECs. LPS, HSL, CpG, pili and flagellin had no effect on sPLA2-IIA expression and only flagellin induced IL8 secretion by these cells ( Fig. 5e , Supplementary Fig. 7f ). Interestingly, the PAK mutant Δpsc F, lacking the type-3 secretion system (T3SS), induced sPLA2-IIA expression at much lower levels compared with the parent strain PAK ( Fig. 5f ). In contrast, the T2SS mutant (Δ xcp Q) induced this expression at similar levels compared with PAK ( Fig. 5f ). Deletion of T3SS but not T2SS increased IL8 secretion compared with parent strain ( Supplementary Fig. 8a ). In subsequent studies, the effect of PA and SA on sPLA2-IIA expression was examined in pBECs isolated from CF patients. As observed in IB3-1 cells, PAK strain induced significant sPLA2-IIA production by pBECs, whereas SA Newman strain had no effect on this production ( Fig. 5g ). Here again, the T3SS-deficient strain induced sPLA2-IIA production at lower levels compared with parent PAK wild-type strain, but induced similar IL8 secretion ( Fig. 5g , Supplementary Fig. 8b ). PAK strain of PA is known to inject three different toxins (ExoS, ExoT and ExoY) into host cells through T3SS (ref. 29 ). Thus, the identification of T3SS as the virulence factor inducing sPLA2-IIA expression by PA allowed us to search which toxin mediated this expression. Our findings showed that among the toxins, ExoS played a key role in sPLA2-IIA expression. Indeed, the ExoS-deficient mutant of PAK (Δ exoS ) induced much lower sPLA2-IIA expression in IB3-1 cells ( Fig. 5h ), but induced higher IL8 secretion ( Supplementary Fig. 8c ) compared with the parent strain and the mutants deficient for other toxins ExoT (Δ exoT ) and ExoY (Δ exoY ). ExoS is a bifunctional toxin displaying two enzymatic domains: GTPase-Activating Protein (GAP) and ADP-ribosyltransferase (ADPRT) [30] . To distinguish which enzymatic domain was involved in sPLA2-IIA expression, we used the PA strain PA103Δ exoU Δ exoT in which a plasmid containing wild-type or mutant of ExoS toxin has been introduced [31] . Our data showed that the ExoS toxin lacking ADPRT (ADPRT − ), but not GAP activity (GAP − ), failed to induce sPLA2-IIA expression compared with the wild-type toxin (ExoS + ; Fig. 5i ). KLF2 is a key factor in ExoS-induced sPLA2-IIA expression We finally investigated the signalling pathways by which ExoS induced sPLA2-IIA expression in IB3-1 cells. Our studies showed that pharmacological inhibition of NF-κB (MG-132 inhibitor) and AP-1 (SR-11302 inhibitor) had no effect on PAK-induced sPLA2-IIA expression ( Fig. 6a ) but decreased IL8 secretion induced by PA ( Supplementary Fig. 8d ). This prompted us to pursue other transcription factors that could be involved in ExoS-induced sPLA2-IIA expression. Krüppel-Like Factor 2 (KLF2) is a transcription factor known to be induced by bacterial toxins and to modulate host immune functions [32] . Our results showed that PAK stimulated KLF2 expression in IB3-1 cells and that deletion of ExoS from PAK strain markedly reduced this expression ( Fig. 6b ). However, deletion of ExoT and ExoY had no effect on KLF2 expression ( Fig. 6b ). Interestingly, gene silencing of KLF2 in IB3-1 cells decreased PAK-induced sPLA2-IIA expression ( Fig. 6c,d ). 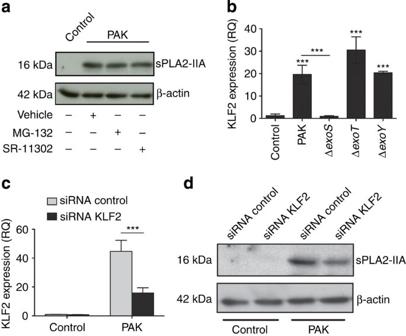Figure 6: ExoS-induced KLF2 factor is involved in sPLA2-IIA expression. (a) Western blot showing the effect of NF-κB (MG-132, 3 μM) and AP-1 (SR-11302, 1 μM) inhibition on sPLA2-IIA expression in IB3-1 cells. (b) KLF2 expression in IB3-1 cells after infection with PAK and toxin-deficient strains ExoS (ΔexoS), ExoT (ΔexoT) and ExoY (ΔexoY). mRNAs were collected after 3 h of infection and KLF2 expression was quantified by RT-qPCR. (c) Silencing of KLF2 expression by specific pool of siRNA (siRNA KLF2) quantified by RT–qPCR, compared with non-specific siRNAs (siRNA Control). (d) Western blot analysis of sPLA2-IIA expression in PAK-infected IB3-1 cells after KLF2 silencing using siRNA. Cells treated by non-specific (siRNA Control) or KLF2 siRNA (siRNA KLF2) were infected by PAK strain for 1 h and protein was collected 24 h later for immunoblotting. Data inbandcwere presented as mean±s.e.m. from at least three independent experiments. ***P<0.001 determined by one-way analysis of variance, followed by Bonferroni multiple’s comparisons test. Immunoblots shown were representative results from at least three independent experiments. Full blots are available inSupplementary Fig. 9. Figure 6: ExoS-induced KLF2 factor is involved in sPLA2-IIA expression. ( a ) Western blot showing the effect of NF-κB (MG-132, 3 μM) and AP-1 (SR-11302, 1 μM) inhibition on sPLA2-IIA expression in IB3-1 cells. ( b ) KLF2 expression in IB3-1 cells after infection with PAK and toxin-deficient strains ExoS (Δ exoS ), ExoT (Δ exoT ) and ExoY (Δ exoY ). mRNAs were collected after 3 h of infection and KLF2 expression was quantified by RT-qPCR. ( c ) Silencing of KLF2 expression by specific pool of siRNA (siRNA KLF2) quantified by RT–qPCR, compared with non-specific siRNAs (siRNA Control). ( d ) Western blot analysis of sPLA2-IIA expression in PAK-infected IB3-1 cells after KLF2 silencing using siRNA. Cells treated by non-specific (siRNA Control) or KLF2 siRNA (siRNA KLF2) were infected by PAK strain for 1 h and protein was collected 24 h later for immunoblotting. Data in b and c were presented as mean±s.e.m. from at least three independent experiments. *** P <0.001 determined by one-way analysis of variance, followed by Bonferroni multiple’s comparisons test. Immunoblots shown were representative results from at least three independent experiments. Full blots are available in Supplementary Fig. 9 . Full size image Chronic bacterial infections of CF airways, in addition to recurrent lung inflammation, are major causes of morbidity and mortality of CF patients. In most cases, SA colonizes airways of young CF patients, while PA predominates in those of adult patients [10] , [11] , [12] . A number of hypotheses have been proposed to explain the elimination of SA from airways of CF patients [33] , [34] , [35] , [36] . However, the pertinence of these hypotheses remained elusive, probably due to the complexity of CF infection and the lack of relevant animal models. The present work suggests that sPLA2-IIA, a host enzyme endowed with potent bactericidal activity, participates in SA elimination from CF airways. We showed the presence of this enzyme in CF expectorations and an increase of its levels with the age of patients. We also demonstrated that sPLA2-IIA levels in CF expectorations were sufficient to kill SA without significant effect on PA. We suggest that PA infection enhances sPLA2-IIA production, which in turn participate to SA elimination in CF airways. The apparent age-related increase of sPLA2-IIA levels in CF expectorations was dissociated from the evolution of airways inflammation of CF patients. In contrast to sPLA2-IIA levels, those of cytokines did not increase with the age of the patients. This might be explained by the fact that both SA and PA induced airway inflammation, whereas only PA stimulated sPLA2-IIA production. Although it is not possible to establish a direct causal relationship between sPLA2-IIA levels and PA infection in CF expectorations, our studies with animal models and cell cultures suggest a role for PA in the induction of sPLA2-IIA production in CF airways. Thus, the observed age-dependent increase of sPLA2-IIA levels in CF expectorations is likely due to the progressive airways infection by PA rather than to the age of patients. Our in vitro studies are in agreement with the dissociation between inflammation and sPLA2-IIA expression. Indeed, flagellin from PA efficiently induced IL8 production, but did not stimulate sPLA2-IIA expression by BECs. Moreover, compared with the PAK parent strain, the T3SS (Δ pscF ) and ExoS (Δ exoS ) mutants were less efficient in inducing sPLA2-IIA expression but stimulated significantly IL8 production. In addition, SA isolates from CF patients induced IL6 production with a higher potency compared to PA isolates, but failed to stimulate sPLA2-IIA expression in BECs. These findings suggest that sPLA2-IIA expression and cytokine production are probably induced by different mechanisms in CF airways. Although sPLA2-IIA has been shown to kill preferentially Gram-positive compared with Gram-negative bacteria [17] , [37] , the bactericidal effect of this enzyme on clinical isolates collected from infected CF patients have been poorly investigated. Previous studies showed that rhsPLA2-IIA was able to kill SA and PA clinical isolates collected from CF patients with almost similar efficiency [38] . However, in those studies, high (non-physiological) rhsPLA2-IIA concentrations (>8 μg ml −1 ) have been used thus making it difficult to examine the selectivity of rhsPLA2-IIA action on SA versus PA isolates. In the present work, we used concentrations of rhsPLA2 ranging from 10 ng ml −1 to 10 μg ml −1 , which allowed us to establish the discriminative action of sPLA2-IIA on SA compared with PA isolates. The results showed that sPLA2-IIA concentrations from 10 to 100 ng ml −1 (which are close to those detected in CF expectorations) were able to kill almost all SA isolates. However, PA isolates are resistant to sPLA2-IIA action even to 10 times higher concentrations. It should also be mentioned that laboratory strains and clinical isolates of SA were killed at similar sPLA2-IIA concentrations suggesting that the bacterial phenotypic changes occuring in CF airways, with chronic infection, does not modify the sensitivity of these bacteria to sPLA2-IIA action. Our studies showed that although sPLA2-IIA is detected in most of CF expectorations, SA is still present in some expectorations. It is likely that the sPLA2-IIA levels in airways of certain CF patients are not sufficient to totally eliminate SA. It is also possible that part of SA colonies in CF airways resist somehow to sPLA2-IIA action. Indeed, Koprivnjak et al. [39] previously showed that mutation of SA wall teichoic acid conferred resistance to sPLA2-IIA activity. A number of direct and indirect evidences of the present work suggest that PA promotes SA elimination from airways via a sPLA2-IIA-dependent mechanism. Indeed: (i) PA but not SA infection, induced sPLA2-IIA expression in lungs and isolated airways epithelial cells, (ii) sPLA2-IIA killed SA much more efficiently than PA both in vitro and in animal models of coinfection by these bacteria, (iii) airways produced sPLA2-IIA in response to PA infection to promote the killing of SA and/or alteration of its membrane integrity. In these studies, almost identical findings were observed with either laboratory strains or clinical isolates of PA and SA. The sPLA2-IIA bactericidal role was also supported by the fact that transgenic mice overexpressing human sPLA2-IIA cleared more efficiency SA than PA and exhibited higher survival compared with their littermates after pulmonary infection with SA but not PA. In agreement with this capacity, a sPLA2-IIA inhibition increased guinea pigs mortality by pulmonary coinfection with PA and SA. Our studies showed that BECs, known to play a key role in CF pathogenesis, are a major cell source of sPLA2-IIA in CF airways. Indeed, we observed a marked positive staining of sPLA2-IIA in airway epithelial cells in all sections of bronchial explants from CF patients at significantly higher intensity compared with non-CF bronchial explants. The sPLA2-IIA staining was also detected in infiltrating neutrophils. Similar observation has been previously reported, but this remained controversial [40] , [41] . sPLA2-IIA is stored in granules of neutrophils but this may also reflect the phagocytosis of extracellular sPLA2-IIA associated with bacteria. It was not possible to obtain explants from non-infected CF patients to assay whether increased sPLA2-IIA expression resulted from CFTR mutation and/or PA infection. However, our in vitro studies showed that sPLA2-IIA was not constitutively expressed in pBECs from CF and non-CF patients. This expression increased after PA infection but its levels remained similar in CF and non-CF pBECs. This suggested that CFTR mutations have no effect on sPLA2-IIA expression that is clearly induced by PA infection ( Fig. 5d ). We propose that in CF context, CFTR mutations facilitated PA airways colonization, which in turn induced sPLA2-IIA expression by host cells. These data contrasted with those of our previous studies with cell lines in which we showed that CF cell lines produced more sPLA2-IIA than non-CF cell lines either at baseline or after stimulation [42] . This is not surprising as, in general, cell lines are known to differ markedly from corresponding primary cells in their metabolism and response to exogenous stimuli. We identified for the first time the T3SS as a major virulence factor involved in this induction. The T3SS is a secretion apparatus used by PA to inject effector proteins into host cells and to establish infection [43] . It allows injection of toxins (ExoS/T/Y/U) endowed with different biological activities that interfere with a number of signalling pathways of host cells [30] ). Interestingly, it has been shown that T3SS expression is lost in chronically infected CF patients [13] , [29] . However, other studies reported that up to 29–41% of PA strains from chronically infected CF patients still expressed the T3SS (refs 44 , 45 ). In addition, exoS gene was detected in all PA isolates from CF patients examined. Our work also highlighted the role of KLF2 transcription factor in PA-induced sPLA2-IIA expression. This transcription factor, also called lung KLF, belongs to the SP-1 zinc-finger transcription factor [46] . KLF2 exerts an anti-inflammatory activity in endothelial cells, monocytes and epithelial cells [47] , [48] , [49] . Our studies report for the first time the implication of a transcription factor of the KLF family in sPLA2-IIA transcription. In line with our results, PA infection of CF BECs increased KLF2 expression in an ExoS-dependent manner [32] . Other bacterial species also enable to induce KLF2 expression [50] , [51] . Although the mechanism by which ExoS induces KLF2 expression is still unclear, our studies suggest that this induction is independent of RhoA, a potential target suggested by others [50] . Indeed, ExoS is a bifunctional toxin with two enzymatic domains, GAP and ADPRT [30] , and only the GAP domain is responsible of RhoA inactivation [52] . Our data showed that the ADPRT, but not the GAP domain, is involved in ExoS-induced sPLA2-IIA expression. In addition, deletion of ExoT, which also displays GAP domain, failed to modulate sPLA2-IIA expression. Although the mechanisms that may explain the inability of SA to induce sPLA2-IIA expression are still unknown, it is clear that this inability was not due to a failure of this bacterium to stimulate host cells. Indeed, at multiplicity of infection that fully stimulated cytokines production, SA was unable to induce sPLA2-IIA expression by BECs. It remains to be investigated whether the inability to stimulate sPLA2-IIA expression is a general property of Gram-positive bacteria. Given that Gram-positive bacteria are in general highly sensitive to sPLA2-IIA bactericidal effects (compared with Gram-negative bacteria), the inability to induce the production of sPLA2-IIA by Gram-positive bacteria may represent an evolutionary adaptation to escape sPLA2-IIA bactericidal action and to colonize the host. In conclusion, our findings suggest that sPLA2-IIA participates to the progressive elimination of SA from CF airways. We propose that PA colonization improves this elimination by increasing sPLA2-IIA expression of airways cells. In agreement, previous studies showed that sPLA2-IIA is present in human and animal biological fluids or cell supernatants at sufficient levels to kill bacteria [21] , [53] , [54] , [55] , [56] . AMPs such as LL-37 have also been shown to play a role in pulmonary host defense toward SA and PA in CF lungs [57] , although the antimicrobial activity of these AMPs is impaired in CF airways [57] , [58] , [59] . In addition, to our knowledge among all AMPs and sPLA2s reported in the literature, sPLA2-IIA displays the most potent and selective bactericidal action toward Gram-positive bacteria, such as SA. We should, however, keep in mind that, in addition to sPLA2-IIA, other processes might also potentially contribute to the age-dependent decrease of SA loads in CF airways [33] , [34] , [35] , [36] . Thus, sPLA2-IIA can be considered as a part of complex process involved in the selective elimination of SA from CF airways. Most importantly, the present work indicates that one bacterium can kill another one by manipulating the innate immunity of the host. This opens a new area of research to investigate the role of host antimicrobial molecules in the dynamic of microbiota. Bacterial preparations PA strains PAO1, CHA, PAK WT and PAK mutants Δ mucA , Δ pscF and Δ xcpQ were kindly provided by Dr Reuben Ramphal (University of Florida, Gainesville, FL, USA). Professor Eric Pearlman (Case Western Reserve University, Cleveland, OH, USA) kindly provided PAK WT, Δ exoS , Δ exoT and Δ exoY strains. PA103 Δ exoU Δ exoT supplemented with pUCP empty vector or containing gene encoding for ExoS WT toxin or mutants (ADPRT − , GAP − and ADPRT − /GAP − ) [31] were kindly provided by Dr Joan C. Olson (West Virginia University, Morgantown, WV, USA). All SA strains used in this study were kindly provided by Dr Tarek Msadek (Institut Pasteur, Paris, France). Clinical isolates of PA and SA were collected from CF patients (Hôpital Cochin, Paris, France). All the tested PA clinical isolates were positive for exoS gene, detected by quantitative PCR (qPCR) on genomic DNA using the following primers (F: 5′-AGAGAGCGAGGTCAGCAGAG-3′ and R: 5′-AGGCGTACATCCTGTTCCTG-3′). PAK strain ( exoS + ) and PA103 ( exoS − ) were used as positive and negative control, respectively [60] . In the present studies, PA PAK strain and SA Newman strain were used unless mentioned in the text. Bacteria were prepared as described previously [61] , [62] . In brief, a single colony was grown overnight in LB medium with agitation at 37 °C. The cultured bacterial suspension was further diluted in fresh LB and grown again to reach mid-log phase. After centrifugation (3,000 g , 15 min at 25 °C), bacterial pellet was rinsed and suspended in appropriate volume of PBS. The bacterial concentrations were calculated according to OD value measured at 600 nm and further adjusted to the approximate desired concentration for in vitro or in vivo experiments. Cell culture and bacterial infection Human bronchial epithelial IB3-1 cell line bearing CF mutant F508del/W1282X genotype [28] , and primary BECs (pBECs) collected from different CF and non-CF patients and commercially available at Epithelix (Geneva, Switzerland) were used in the studies. IB3-1 cells cultured in LHC-8 medium (Cat. No. 12678-017, Invitrogen) were seeded in culture dish and incubated with PA and SA (WT and mutants). The plates were centrifuged (500 g , 25 °C, 5 min) to initiate the infection. One hour later, cells were rinsed three times with prewarmed culture medium containing tobramycin (40 μg ml −1 ) to kill extracellular bacteria and then incubated for additional 24 h in the presence of antibiotic before collecting cells. Pathogen-associated molecular patterns preparations of PA (kind gift of Dr Reuben Ramphal, University of Florida, Gainesville, FL, USA) were also incubated with cells for 24 h in the presence of antibiotic. pBECs isolated from CF patients carrying homozygous F508del mutation or from non-CF subjects, were from Epithelix (Geneva, Switzerland) and cultured in MucilAir culture medium (Epithelix) in transwell with air–liquid interface. The cells were infected with bacteria at the apical side for 3 h and then bacteria were removed by rinsing and incubated with PBS–tobramycin (40 μg ml −1 ) for 30 min followed by incubation of the apical pole in air–liquid interface for additional 24 h. In certain experiments, inhibitor of proteasome/NF-κB (MG-132, 3 μM, Cat. No. 474791, Calbiochem, MA, USA) or inhibitor of AP-1 (SR-11302, 1 μM, Cat. No. 2476, Tocris, CA, USA) were added 1 h before infection with bacteria and maintained for overnight incubation. After reaction, cell-free culture medium was kept at −80 °C for further analysis. Cells were collected for analysis of protein expression (human sPLA2-IIA) using western blot (see protocol below). IL8 levels in supernatant of culture medium were examined by enzyme-linked immunosorbent assay (ELISA; CXCL8/IL8 Duoset, Cat. No. DY208, R&D systems, MN, USA). Cell cytotoxicity was controlled using lactate deshydrogenase assay (Promega, France) in the culture medium. RNA interference in IB3-1 cells Non-specific small-interfering RNA (siRNA) (ON-TARGETplus non-targeting control pool, Cat. No. D-001810-10-05) and KLF2 siRNA (smartpool ON-TARGETplus KLF2 siRNA, Cat. No. L006928-00-0005) were commercially available from Dharmacon (Fisher Scientific, Illkirch, France). Subconfluent IB3-1 cells were transfected with siRNA (100 nM) using Lipofectamine 2000 (1.5 μg ml −1 , Invitrogen) for 8 h, before complete medium (LHC-8 supplemented with 5% fetal calf serum and penicillin/streptomycin 100 U ml −1 each) was added. Twenty-four hours after transfection, cells were incubated in antibiotic- and serum-free LHC-8 medium until infection. In vitro killing studies Recombinant human sPLA2-IIA (rhsPLA2-IIA, prepared by Dr Gerard Lambeau, Université de Nice Sophia Antipolis, Sophia Antipolis, Valbonne, France) was used in the present studies. Bacteria (10 5 c.f.u. ml −1 ) were incubated with or without rhsPLA2-IIA in the reaction buffer (0.1 M Tris pH8.0, 1 mM CaCl 2 and 0.1% fatty acid-free bovine serum albumin (BSA)) at 37 °C. Two hours later, bacterial suspension was serially diluted with PBS and aliquots were streaked on LB-agar plate and incubated 24 h at 37 °C. Bactericidal effect of rhsPLA2-IIA was checked by counting bacterial colonies on the plates and expressed as percentages of c.f.u. compared with that of treatment without sPLA2-IIA. In certain experiment, recombinant protein was preincubated with its specific inhibitors, YM26734 (10 μM, Cat. No. 2522, Tocris, CA, USA), RO032007A (10 μM, kind gift of Pr. Michael Gelb, University of Washington, Seatlle, WA, USA) [22] or specific neutralizing antibody (10 μg ml −1 , prepared by Dr Gerard Lambeau) [23] for 30 min before incubation with bacteria. Bacterial membrane hydrolysis analysis Bacteria were prepared as described above except that next morning diluted bacterial suspension was grow to mid-log phase in the presence of 3 H-oleic acid ( 3 H-OA) (Cat. No. NET289, NEN Radiochemicals, MA, USA). This allowed labelling of bacterial membrane phospholipids [55] . After centrifugation (3,000 g , 25 °C, 15 min), bacterial pellets were suspended in 5 ml of LB medium and incubated for additional 30 min to allow binding oleic acid on the surface of bacteria to be incorporated, followed by rinsing once using 0.15 M NaCl to remove non-incorporated 3 H-OA. The desired inoculum (10 8 c.f.u. ml −1 per reaction) suspended in assay buffer (0.1 M Tris pH8, 1 mM CaCl 2 and 0.1% fatty acid-free BSA) was then incubated for 2 h at 37 °C with rhsPLA2-IIA (from 10 to 100 ng ml −1 ), BALFs from bacteria-infected guinea pigs (see protocol below) or supernatants of sputum from CF patients (see protocol below). After reaction, the released free 3 H-OA in supernatant (centrifugation at 13,000 g for 1 min) was monitored using scintillation counting. The levels of 3 H-OA contained in aliquots of bacterial suspension or centrifuged supernatant from control groups (bacteria were incubated with PBS), were defined as total and blank (non-specific) count, respectively. In certain experiments, samples were pretreated with the sPLA2 inhibitor YM26734 (10 μM) for 30 min before incubation with bacteria. The results were presented as percentage of released free 3 H-OA from total incorporated 3 H-OA by bacteria. Studies of airways bacterial clearance and animal survival Animals were housed in the Institut Pasteur animal facilities accredited by the French Ministry of Agriculture for performing experiments on live rodents. Work on animals was performed in compliance with French and European regulations on care and protection of laboratory animals (EC Directive 2010/63, French Law 2013-118, February 6th, 2013). All experiments were approved by the Institut Pasteur’s Ethics Committee #89 and registered under the reference 2014–0014. Transgenic mice overexpressing human sPLA2-IIA (sPLA2-IIA-Tg) were from Taconic (Denmark) and generated by inserting 6.2 kb full length of human sPLA2-IIA gene into mouse genome and bred to c57BL/6 mouse [25] . The corresponding littermates (sPLA2-IIA-Wt) with c57BL/6 genetic background were natural sPLA2-IIA-deficient mouse due to frameshift mutation of this gene [63] . Mice (males and females, 7–9 weeks) were bred in our animal facility and infected intratracheally with PA and/or SA (10 6 , 10 7 , 10 8 or 10 9 c.f.u.) suspended in 50 μl of PBS as indicated in legend. Mice mortality was monitored up to 180 h. In certain experiments, 6 or 24 h after infection with PA and/or SA, lung homogenates were prepared as described previously [64] and bacterial loads in the lung were examined by checking bacterial c.f.u. in lung homogenates on LB-agar plate. The bacterial loads in the lung were expressed as c.f.u. ml −1 lung homogenate. Male Hartley guinea pigs (~2–3 weeks old, 150 g, purchased from Charles River, France) were also infected by PA and/or SA (suspended in 100 μl of PBS) in this study. Bacterial load in the lungs were evaluated by checking bacterial c.f.u. in BALs 24 h after infection. In some experiments, 24 and 1 h before bacterial infection, 50 μl of the sPLA2 inhibitor YM26734 (2 mg kg −1 body weight, 4 mM in dimethylsulphoxide) or vehicle (dimethylsulphoxide) were introduced by intravenous injection and the third dose was given by intratracheal instillation together with bacterial preparations. Animal survival was monitored for 24 h. sPLA2 activity in BALF was examined 24 h after infection. For killing assay with lung homogenates, 100 μl of PBS or LPS (300 μg kg −1 body weight) were instillated intratracheally to guinea pigs. Twenty-four hours later, lungs were collected and homogenized in PBS using Lysing matrix D (MPbiomedicals, Illkirch, France). Then, 90 μl of lung homogenates were incubated with bacteria (10 5 ml −1 ) in reaction buffer (0.1 M Tris pH8, 1 mM CaCl 2 and 0.1% fatty acid-free BSA) for 2 h, before c.f.u. counting by streaking on agar plates. When indicated, homogenates were pretreated with the sPLA2 inhibitor YM26734 (10 μM) for 30 min before incubation with bacteria. Sputum treatment All sputum samples from CF patients were collected in accordance with the guidance of European Union and the local Committees on Human Research CPP Ile-de-France 1 and registered under the reference 2013-Nov.-13406. Informed consent was obtained for all patients. We did not share personal information of patients according to privacy policy. The collected sputum was firstly diluted in PBS (1:1 vol) and homogenated with repeated vigorous agitation. To decrease the viscosity of samples due to large amounts of DNA and F-actin present in expectorations [65] , [66] , an aliquot (200 μl) of mixed suspension was treated with recombinant bovine DNase I (10 units, Roche) for 1 h at 37 °C with up–down rotation. After reaction, the supernatants were collected by centrifugation (14,000 g at 4 °C for 10 min) and further irradiated in dry ice using a 137 Cs-source γ-irradiator (IBL 637, CIS bio international) to kill bacteria in sputum, which was verified by streaking aliquot of sample on LB-agar plate and checking bacterial colonies. The samples were then kept at −80 °C for further analysis. sPLA2 activity and EIA assay The sPLA2 activity in BALF as well as supernatants of expectorations was measured using 3 H-OA-labelled E. coli membrane phospholipids as substrate [67] , [68] . In brief, aliquots of BALFs or supernatants of expectorations (1–10 μl) were incubated with 10 μl substrate (containing around 6,000 c.p.m.) at 37 °C in assay buffer (0.1 M Tris pH7.5, 1 mM CaCl 2 , 0.2% sodium azide) with 200 μl of total volume. Thirty minutes later, the reactions were stopped by adding 100 μl of stop buffer (0.25% BSA in assay buffer, pH7.5) followed by centrifugation (1,800 g at 4 °C for 10 min). The sPLA2 activity was presented as percentage of radioactivity in the supernatant compared with that of total count (defined as radioactivity detected in mixed suspension of substrate incubated with PBS). The specificity of this activity assay was verified in the presence of selective sPLA2 activity inhibitor, YM26734 (10 μM), which was preincubated with sample for 30 min before adding substrate. The quantification of specific sPLA2-IIA protein in the patients’ expectoration was performed using a commercial enzyme immunoassay kit (EIA kit, Cat. No. 585000, Cayman Chemical, MI, USA) according to manufacturer’s instruction. Analysis of sPLA2-IIA and KLF2 expression and cytokines TNFα, KC and IL6 levels in BALFs of sPLA2-IIA-Wt and sPLA2-IIA-Tg mice were measured with mouse TNF-alpha DuoSet (Cat. No. DY410), mouse CXCL1/KC DuoSet (Cat. No. DY453) and mouse IL6 DuoSet (Cat. No. DY406) ELISA kits from R&D Systems, respectively. IL8 secretion in cell-free culture medium from human CF epithelial IB3-1 cells, basal pole medium of primary epithelial cells and supernatant of patients’ sputum, was examined using commercial kit human CXCL8/IL8 DuoSet (Cat. No. DY208) from R&D systems (MN, USA). IL6 and IL1β production were also examined in some experiments using human IL6 DuoSet (Cat. No. DY206) and human IL1 beta/IL1-F2 DuoSet (Cat. No. DY201) ELISA kits from R&D system. sPLA2-IIA expression in these human cells was analysed by western blot. In brief, total proteins were extracted from IB3-1 and pBECs after incubation with bacteria or bacterial pathogen-associated molecular patternss preparations. After SDS-polyacrylamide gel electrophoresis and transfer to polyvinylidene fluoride membrane, human sPLA2-IIA expression was analysed by immunoblot using anti-human sPLA2-IIA polyclonal antibody (1 μg ml −1 , Cat. No. Ab47105, Abcam, MA, USA). Original full scans are presented in Supplementary Fig. 9 . Total RNA was extracted from IB3-1 cells using RNeasy mini kit (Qiagen, CA, USA) according to manufacturer’s instruction. The expression of KLF2 was analysed by qPCR using 7900HT fast real-time PCR system (Applied Biosystems). The primers used for qPCR were GAPDH (F: 5′-AGGGCTGCTTTTAACTCTGGT-3′, R: 5′-CCCCACTTGATTTTGGAGGGA)-3′ and KLF2 (F: 5′-CCTCCCAAACTGTGACTGGT-3′, R: 5′-ACTCGTCAAGGAGGATCGTG-3′). The qPCR was performed using SYBR green master mix. The results are presented as relative quantification of gene expression using the 2 −ΔΔCT method. Human lung tissues Human lung tissues were obtained from nine non-smoking CF adults at transplantation and from 10 non-smoking Controls undergoing lung resection for peripheral lung cancer. Informations about infectious status of CF patients are provided in Supplementary Table 1 . Lung tissue samples were fixed in 10% neutral buffered formalin by inflation immersion and embedded in paraffin. Studied locations were chosen randomly. The study conformed to the Declaration of Helsinki and all to the rules of the local Committees on Human Research CPP Ile-de-France 1 and registered under the reference 2013-Nov.-13406. Informed consent was obtained for all patients. Immunohistochemical staining and morphometric analysis Immunohistochemical staining was performed on 5 μm paraffin-embedded sections. The sections were deparaffinized, rehydrated and treated with 0.3% H 2 O 2 in methyl alcohol [69] . The primary antibody (Ab) raised against sPLA2-IIA was a rabbit polyclonal Ab (4 μg ml −1 , Cat. No. Ab23705, Abcam, MA, USA) and was diluted in PBS containing 0.05% Tween-20 and 1% BSA. Antigen unmasking by incubation with target retrievial solution RTU (Dako) for 40 min was required to improve the quality of staining. Biotinylated anti-rabbit Ab (1:200; Vector Laboratories, Burlingame, CA, USA) was used for secondary Ab, and bound Ab were visualized according to standard protocols for avidin–biotin–peroxidase complex method (Elite ABC kit; Vector Laboratories). Tissue sections were counterstained with haematoxylin. Omission of primary Ab and incubation with irrelevant immunoglobulins were used as negative controls. Quantification of sPLA2-IIA epithelial immunostaining was performed by point counting using a grid [70] . Points within the grid falling on epithelial cells staining positively were counted. Volume occupied by sPLA2-IIA positively-stained cells in epithelium was expressed per volume of epithelium. Analysis was performed on at least 20 randomly chosen high-magnification ( × 400) photomicrographs. Statistical analysis The results were presented as mean±s.e.m. and the data were analysed using statistic software GraphPad Prism 5.0. The level of statistical significance was determined either by Student’s t -test, one-way analysis of variance (Newman–Keuls multiple comparisons test or Bonferroni multiple comparisons test) or two-way analysis of variance. Survival studies were analysed by Log-rank test. How to cite this article: Pernet, E. et al. Pseudomonas aeruginosa eradicates Staphylococcus aureus by manipulating the host immunity. Nat. Commun. 5:5105 doi: 10.1038/ncomms6105 (2014).